Image transmission through an opaque material Optical imaging relies on the ability to illuminate an object, collect and analyse the light it scatters or transmits. Propagation through complex media such as biological tissues was so far believed to degrade the attainable depth, as well as the resolution for imaging, because of multiple scattering. This is why such media are usually considered opaque. Recently, we demonstrated that it is possible to measure the complex mesoscopic optical transmission channels that allow light to traverse through such an opaque medium. Here, we show that we can optimally exploit those channels to coherently transmit and recover an arbitrary image with a high fidelity, independently of the complexity of the propagation. In a classical optical system, the propagation of a complex field from one plane to another is well understood, be it by Fresnel or Fraunhofer diffraction theory, or by ray tracing for more complex cases [1] . However, all these approaches break down when multiple scattering occurs [2] . A medium in which light is scattered many times mixes all input wavevectors in a seemingly random way, and is usually considered opaque. Until recently, scattering has always been considered as noise [3] , and most imaging techniques in turbid media rely on ballistic photons only [4] , [5] , which prevents the study of thick scattering samples. Following works in acoustics [6] , recent experiments have demonstrated that multiply scattered light can nonetheless be harnessed, thanks to wavefront control [7] , [8] , [9] , and even put to profit to surpass what one can achieve within a homogenous medium in terms of focusing [10] . In our experiment (see Fig. 1 ), we illuminate an object with a laser (displayed through a spatial light modulator (SLM)), and recover its image on a charge-coupled device (CCD) camera, after propagation through a thick opaque sample. As expected, we measure on the camera a speckle that bears no resemblance to the original image. This speckle is the result of multiple scattering and interferences in the sample. 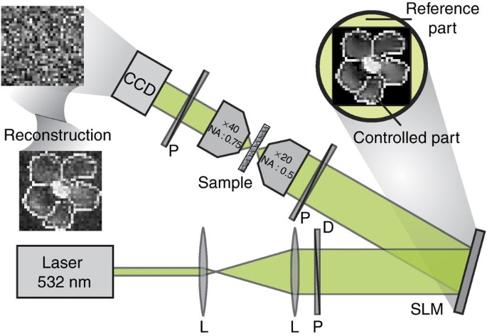Figure 1: Experimental setup. A 532 nm laser is expanded and reflected off a spatial light modulator (SLM). The laser beam is phase-modulated, focused on the multiple scattering sample and the output intensity speckle pattern is imaged by a CCD camera. L, lens; P, polarizer; D, diaphragm. The object to image is synthetized directly by the SLM, and reconstructed from the complex output speckle, thanks to the transmission matrix. Figure 1: Experimental setup. A 532 nm laser is expanded and reflected off a spatial light modulator (SLM). The laser beam is phase-modulated, focused on the multiple scattering sample and the output intensity speckle pattern is imaged by a CCD camera. L, lens; P, polarizer; D, diaphragm. The object to image is synthetized directly by the SLM, and reconstructed from the complex output speckle, thanks to the transmission matrix. Full size image Although it can be described on average by the diffusion equation or Monte Carlo simulation [11] , the propagation through a real linear multiple scattering medium is too complex to be described by classical means. Nonetheless, multiple scattering is deterministic and information is not lost. In other terms, the measured pattern on the CCD is the result of the transmission of light through a large number of very complicated optical channels, each of them with a given complex transmission. Here, we study the inverse problem of the reconstruction of an arbitrary image, and show that it is possible to recover it through the opaque medium. A prerequisite is, however, to measure the so-called transmission matrix (TM) of our optical system. We define the mesoscopic TM of an optical system for a given wavelength as the matrix K of the complex coefficients k mn connecting the optical field (in amplitude and phase) in the m th of M output-free mode to the one in the n th of N input-free mode. Thus, the projection of the outgoing optical field on the m th free mode is given by where is the complex amplitude of the optical field in the n th incoming free mode. In essence, the TM gives the relationship between input and output pixels, notwithstanding the complexity of the propagation, as long as the medium is stable. A singular value decomposition of the TM gives the input and output eigenmodes of the system, and singular values are the amplitude transmission of these modes. Inspired by various works in acoustics [12] , [13] and electromagnetism [14] , we demonstrated in Popoff et al . [15] that it is possible to measure the TM of a linear optical system that comprises a multiple scattering medium. In a nutshell, we send several different wavefronts with the SLM, record the results on the CCD and deduce the TM using phase-shifting interferometry. The singular value distribution of a TM of a homogeneous zone of the opaque sample follows the quarter-circle law (that is, there is no peculiar input/output correlation [16] ), which indicates that light propagation is in the multiple scattering regime with virtually no ballistic photons left. Using this technique, we have access to , where S ref is a diagonal matrix due to a static reference speckle. The input and output modes are the SLM and the CCD pixels, respectively. The measured matrix K obs is sufficient to recover an input image. This TM measurement takes a few minutes, and the system is stationary well over this time. Once the matrix is measured, we generate an amplitude object E obj by subtracting two-phase objects (see Methods for details). A realization takes a few hundred milliseconds, limited only by the speed of the SLM. Here, our aim is to use the TM to reconstruct an arbitrary image through the scattering sample: we need to estimate the initial input E obj from the output amplitude speckle E out . This problem consists in using an appropriate combination of the medium channels and, therefore, using a weighting of singular modes/singular values of the TM matched to the noise and to the transmitted image. Noises of different origins (laser fluctuations, CCD readout noise and residual amplitude modulation) degrade the fidelity of the TM measurement. It is the exact analogue of multiple-input multiple-output information transmission in complex environment that has been studied in the past few years in wireless communications [17] . This inverse problem also bears some similarities to optical tomography [18] , [19] , although in a coherent regime [20] . We show that this allows us to reconstruct the image of an arbitrarily complex object, as viewed through an opaque medium. Reconstruction operators There are two straightforward options. (i) Without noise, a perfect image transmission can be performed by the use of the inverse matrix (or pseudoinverse matrix for any input/output pixels ratio), as , where I is the identity matrix. Unfortunately, this operator is very unstable in the presence of noise. Singular values of are the inverse ones of K obs ; thus, singular values of K obs below noise level result in strong and aberrant contributions. The reconstructed image can hence be unrelated with the input. (ii) In a general case, another possible operator for image transmission is the time reversal operator. This operator is known to be stable regarding noise level, as it takes advantage of the strong singular values to maximize energy transmission [12] . Its monochromatic counterpart is phase conjugation (classically used to compensate dispersion in optics [21] ) and is performed using . has a strong diagonal, but the rest of it is not null, which implies that the fidelity of the reconstruction rapidly decreases with the complexity of the image to transmit [22] . A more general approach is to use a mean square optimized operator (MSO), which we note W . This operator minimizes transmission errors [17] , [23] , estimated by the expected value . For an experimental noise of standard deviation σ on the output pixels, W reads as follows: Without noise, W reduces to the inverse matrix , which is optimal in this configuration, whereas for a very high noise level, it becomes proportional to the transpose conjugate matrix , the phase conjugation operator. It is important to note that σ has the same dimension as and thus has to be compared with the square of the singular values of K obs . Because of this experimental noise, the reconstruction is imperfect. We estimate the reconstruction fidelity by computing the correlation between the image and the object. Improving the reconstruction A general principle is that the reconstruction noise can be lowered by increasing the number of degrees of freedom ( N DOF ) that we measure and control. For a given object corresponding to N input pixels, we investigated two possibilities: averaging over disorder realizations and increasing the number of output modes M . A possible way to average over disorder is to illuminate the object with different wavefronts. It is formally equivalent to transmitting the same image through different channels, as if the image is propagated through different realizations of disorder. To that end, we use different combinations of random phase masks to generate the same 'virtual object' (see Methods). We use this technique to virtually increase N DOF , and we average the results to lower the reconstruction noise. It is the mochromatic equivalent of using broadband signals, which takes advantage of temporal degrees of freedom [24] . 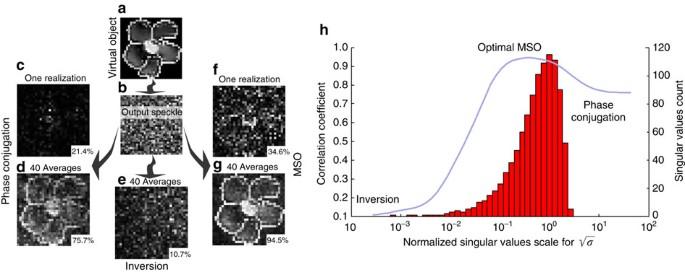Figure 2: Comparisons of the reconstruction methods. (a) Initial greyscale object and (b) a typical output speckle figure after the opaque medium. (c,f) Experimental images obtained with one realization using, respectively, phase conjugation and MSO operator; (d,e,g) experimental images averaging over 40 'virtual realizations' using, respectively, inverse matrix, phase conjugation and MSO operator. Values in insets are the correlation with the objecta. (h) Correlation coefficient betweenEimgandEobjas a function of(line) and singular value distribution ofKobs(bars). Results are obtained averaging over 100 'virtual realizations' of disorder, and bothand singular values share the same scale on the abscissa axis. We show in Figure 2 the results for the image transmission of a greyscale 32 by 32 pixels pattern, and detected on a 32 by 32 pixels region on the CCD. We tested MSO at different noise levels for one realization and for averaging over 40 'virtual realizations' using random phase masks. To find the optimal MSO operator, we numerically compute the optimal σ that maximizes the image reconstruction, hence obtaining an estimation of the experimental noise level. A simple inverse filtering does not allow image reconstruction, even with averaging, whereas phase conjugation converges toward 75% correlated image. In contrast, optimal MSO allowed a 94% correlation for 40 averaging (and a modest 34% correlation in one realization). In addition, optimal MSO is very robust to the presence of ballistic contributions that strongly hinder reconstruction in phase conjugation (see Discussion ). Figure 2: Comparisons of the reconstruction methods. ( a ) Initial greyscale object and ( b ) a typical output speckle figure after the opaque medium. ( c , f ) Experimental images obtained with one realization using, respectively, phase conjugation and MSO operator; ( d , e , g ) experimental images averaging over 40 'virtual realizations' using, respectively, inverse matrix, phase conjugation and MSO operator. Values in insets are the correlation with the object a . ( h ) Correlation coefficient between E img and E obj as a function of (line) and singular value distribution of K obs (bars). Results are obtained averaging over 100 'virtual realizations' of disorder, and both and singular values share the same scale on the abscissa axis. Full size image The second approach to add degrees of freedom is to increase the number M of independent pixels recorded on the CCD. In contrast with focusing experiments in which the quality of the output image depends on the number of input modes N [8] , the quality of image reconstruction depends on the number of output modes M . An important advantage is that the limiting time in our experiment is the number or steps required to measure the TM, equal to 4 N . Thus, we can easily increase M by increasing the size of the image recorded without increasing the measurement time. More than just modifying the N DOF , the ratio γ = M/N ≥1 is expected to change the statistics of the TM. Random matrix theory predicts that for these matrices, the smallest normalized singular value reads . If we increase γ , so does the minimum singular value . In a simple physical picture, recording more information at the output results in picking between all available channels those that convey more energy through the medium. If the energy transported by the most inefficient channel reaches and exceeds the noise level, the TM recording is barely sensitive to the experimental noise. We expect that for an appropriate ratio γ , reaches the experimental noise level. At this point, no singular values can be drowned in the noise and the pseudoinverse operator can be efficiently used. We experimentally recorded the TM for different values of γ ≥1 and tested optimal MSO and pseudoinversion. 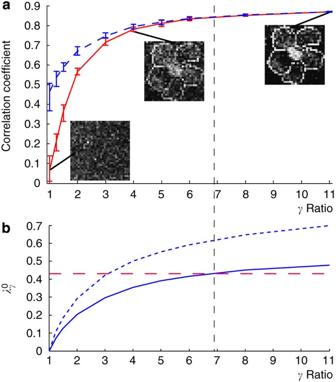Figure 3: Influence of the number of output detection modes. (a) Correlation coefficient betweenEimgand as a function of the asymmetric ratio γ=M/Nof output to input pixels for MSO (dashed line) and for pseudoinversion (solid line), without any averaging. Error bars correspond to the dispersion of the results over 10 realizations. (b) Experimental (solid line) and Marcenko–Pastur16predictions (dashed line) for the minimum normalized singular value as a function ofγ. The horizontal line show the experimental noise level. The results are shown in Figure 3 . Adding degrees of freedom strongly improves the quality of the reconstruction. We see that the quality of the reconstructed image increases with γ and reaches a >85% fidelity for the largest value of γ =11, without any averaging. The minimum singular value also increases with γ . As expected, for , pseudoinversion is equivalent to optimal MSO. One might notice that experimental are always smaller than their theoretical predictions. This deviation can be explained by the amplitude of the reference pattern that induces correlations in the matrix. It is well known in random matrix theory that correlations modify the singular value decomposition of a matrix of identically distributed elements [16] . Figure 3: Influence of the number of output detection modes. ( a ) Correlation coefficient between E img and as a function of the asymmetric ratio γ= M/N of output to input pixels for MSO (dashed line) and for pseudoinversion (solid line), without any averaging. Error bars correspond to the dispersion of the results over 10 realizations. ( b ) Experimental (solid line) and Marcenko–Pastur [16] predictions (dashed line) for the minimum normalized singular value as a function of γ . The horizontal line show the experimental noise level . Full size image So far, we tested image transmission in the case of a homogeneous medium, but what would be the results in more complex conditions ? Here, we study the robustness of this technique in the presence of ballistic contributions, that is, a fraction of light that has not been scattered at all. The singular values of K obs are proportional to the amplitude transmitted through each channel of the system. Ballistic contributions should give rise to strong singular values, corresponding to the apparition of channels of high transmission. These are not spatially homogeneously distributed in energy, contrarily to multiply scattered contributions. Phase conjugation maximizes energy transmission in channel of maximum transmission [12] . Therefore, ballistic high singular values contributions should be predominant in phase conjugation, independent of the image E obj , and will not efficiently contribute to image reconstruction. MSO should not be affected, as it reaches the optimum intermediate between inversion, which is stable except for singular values below noise level, and phase conjugation, which forces energy in maximum singular value channels. In other words, MSO will lower the weight of channels that do not efficiently contribute to the image reconstruction. To experimentally study this effect, we moved the collection objective closer to the sample on a thinner and less homogeneous region, where some ballistic light could be recorded. 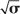Figure 4: Influence of the transmission channels on the reconstruction correlation coefficient betweenEimgandEimgas a function of(line) and singular value distribution ofKobswith ballistic contributions in the transmission matrix, averaged over 100 'virtual realizations' of disorder. Bothand singular values share the same scale on the abscissa axis. High singular value ballistic contributions (highlighted by the black circle) strongly degrade the reconstruction in phase conjugation, whereas MSO is unaffected. We study in Figure 4 the quality of the reconstruction as a function of σ for both experimental conditions (with and without ballistic contributions). Both experiments give comparable results, with 93.6 and 94.5% correlation coefficient, with the optimal MSO operator, and both give very low correlation results for inverse matrix operator. With the phase conjugation operator (equivalent to MSO for high σ ), the experiment sensitive to ballistic contributions give a low correlation coefficient of around 35%, to be compared with the value of 75.7% that we obtained through the multiple scattering sample. This difference can be explained by the presence of a few high singular values contributions (two times greater than the maximum of the other singular values) that perturbate the image reconstruction. Figure 4: Influence of the transmission channels on the reconstruction correlation coefficient between E img and E img as a function of (line) and singular value distribution of K obs with ballistic contributions in the transmission matrix, averaged over 100 'virtual realizations' of disorder. Both and singular values share the same scale on the abscissa axis. High singular value ballistic contributions (highlighted by the black circle) strongly degrade the reconstruction in phase conjugation, whereas MSO is unaffected. Full size image To conclude, we have shown that the TM allows a rapid and accurate reconstruction of an arbitrary image after propagation through a strongly scattering medium (see Supplementary Movie 1 ). Our approach gives a general framework for coherent imaging in complex media, going well beyond focusing and phase conjugation. It is valid for any linear complex media, and could be extended to several novel photonic materials, whatever the amount of scattering or disorder (from complete disorder to weakly disordered photonic crystals [26] , and from superdiffusive [27] to Anderson localization [28] ). The quality of the reconstruction can be increased by harnessing the degrees of freedom of our system, and is very resilient to noise. In addition to its obvious interest for imaging, this experiment strikingly shows that manipulation of wave in complex media is far from limited to single or multipoint focusing. In particular, owing to spatial reciprocity, a similar experiment could be performed using an amplitude and phase modulator by shaping the input wavefront to form an image at the output of an opaque medium, which would allow a resolution solely limited by the numerical aperture of the scattering medium [10] . The main current limitation is the speed of the TM measurement, which is limited only by the SLM. Nevertheless, faster technologies emerge, such as micromirror arrays or ferromagnetic SLMs, that might in the future widen the range of application domains for this approach, including the field of biological imaging. Imaging setup The experimental setup consists of an incident light from a 532 nm laser source (Laser Quantum, Torus) that is expanded, spatially modulated by a SLM (Holoeye, LC-R 2500) and focused on an opaque strongly scattering medium: 80 ± 25 μm-thick deposit of ZnO (Sigma-Aldrich, cat. no. 96479), with a measured transport mean free path of 6 ± 2 μm on a standard microscope glass slide. Polarization optics select an almost phase-only modulation mode [29] of the incident beam, with <10% residual amplitude modulation. The surface of the SLM is imaged on the pupil of a ×10 objective; thus, a pixel of the SLM matches a wave vector at the entrance of the scattering medium. The beam is focused at one side of the sample and the output intensity speckle is imaged on the far side (0.3 mm from the surface of the sample) by a ×40 objective onto a 10-bit CCD camera (AVT Dolphin F-145B). Generation of the amplitude object As there is no simple way to control the amplitude and phase of the incident beam, we generate a virtual amplitude object by substracting two-phase objects. This method is more flexible than placing a real amplitude object in the plane of the SLM. From any phase mask , we could generate a second mask , where the phase of the m th pixel is shifted by . We have with being the j th element of . is proportional to sin and can be estimated by where (resp. ) is the complex amplitude of the output speckle resulting from the input vector (resp. ). How to cite this article : Popoff, S. et al . Image transmission through an opaque material. Nat. Commun. 1:81 doi: 10.1038/ncomms1078 (2010)